Microfluidic probe for single-cell analysis in adherent tissue culture Single-cell analysis provides information critical to understanding key disease processes that are characterized by significant cellular heterogeneity. Few current methods allow single-cell measurement without removing cells from the context of interest, which not only destroys contextual information but also may perturb the process under study. Here we present a microfluidic probe that lyses single adherent cells from standard tissue culture and captures the contents to perform single-cell biochemical assays. We use this probe to measure kinase and housekeeping protein activities, separately or simultaneously, from single human hepatocellular carcinoma cells in adherent culture. This tool has the valuable ability to perform measurements that clarify connections between extracellular context, signals and responses, especially in cases where only a few cells exhibit a characteristic of interest. Cell-to-cell heterogeneity is a feature of processes of great interest in basic and disease research (for example, cancer metastasis [1] , [2] and drug responses of tumour cells [3] , [4] , [5] ). Understanding of these processes can benefit greatly from single-cell measurements, especially those that can relate differences in function or phenotype and the extracellular microenvironment to variations in intracellular state of individual cells [6] , [7] . Traditional cellular assays, however, due to sensitivity limitations, measure average properties of large numbers (usually 10 3 –10 6 ) of cells. Such measurements mask the differences between individual cells [3] , [8] , [9] . Several current techniques allow assaying cells individually for differing types of information. Harnessing nucleic acid amplification and sequencing technologies, a number of assays measure genetic information and gene expression from single cells [10] , [11] , [12] , [13] , [14] . Microfluidic realizations of these assays achieve high sensitivity and throughput. Most such techniques, however, require cells in suspension. Placing adherent cells in suspension destroys information about tissue context, and makes it difficult to relate measured variations to this context or to phenotypic differences observable only when cells are adherent to a substrate. Since even genetically identical cells may respond differently to the same cues [3] , [4] , [5] , as many additional layers of regulation determine cellular behaviour, single-cell measurement at the protein level is desirable. Assaying for protein levels, localization or activity from single cells faces additional challenges over gene-based assays, not only due to the lack of a generic amplification scheme but also because proteins are dynamic on a shorter time scale (and thus more quickly responsive to unwanted perturbations introduced by the assay method). The ability to make measurements of signalling proteins, for example, kinases, at the single-cell level is especially relevant to the major goal of understanding how a cell processes information from external cues to generate a response. This can help in understanding how to alter cell outcomes in a controlled manner, which has great implications for therapeutics [3] , [4] , [5] . Thus a means to obtain a clear picture of signalling events in a cell, and ideally clarify the connection between signalling and phenotype for a particular cell while knowing its external context, is desirable. For examining cell signalling events, protein activity is more relevant than protein level, reporting more directly on actions occurring in the cell. However, levels of proteins and protein post-translational modification (PTM) states, which are less challenging to measure, are often used as proxies for the actual activity. Flow and phospho-flow cytometry, as well as mass cytometry [15] , enable high-throughput multiplexed measurements of these from single cells, but have several drawbacks. A first problem is the assumption that the phosphorylation state of a kinase is a good proxy for its activity. Because of the complex and incompletely understood nature of signalling regulation via phosphorylation (and other protein PTMs), this is not necessarily the case, including for heavily studied kinases such as Akt [16] , [17] , [18] . A corollary issue is that even for cases in which an identified PTM state definitively governs activity level, this can often involve multiple PTMs that are typically not quantified concomitantly [19] . A second challenge is that these assays generally rely on the existence of high-quality antibodies specific for the protein or protein PTM of interest. Third, such assays do not easily permit association of the molecular signalling measurements with a phenotypic characterization of any given cell (other than via surrogate molecular markers), so a goal of ascertaining relationships between signalling state and phenotypic behaviour on a cell-to-cell level is elusive. Finally, these assays, as well as microfluidic approaches to single-cell protein level measurement [20] , predominantly require a suspension step before measurement can be undertaken, which is likely to affect signalling. Direct measurements from single adherent cells, at the genetic or protein level, without perturbing the cells and their extracellular milieu are therefore highly desirable, but limited means currently exist to accomplish this [21] . For the particularly challenging case of measuring protein activities, only a few methods exist, each with its difficulties. Injected sensors present challenges with specificity and stability, and injection disrupts the cell [22] . Live-cell imaging using genetically encoded reporters can provide dynamic information on protein levels and localization or on activity directly [23] , but such reporters are difficult to multiplex, and genetic manipulation presents the risk of affecting the system under study. The approach is also highly resource-intensive, and presents challenges in obtaining quantitative measurements [24] . We have previously used a microfluidic concentrator device to fluorescently monitor specific kinase activities from unfractionated cell lysates using peptide sensors incorporating the non-natural amino acid Sox, a chelation-enhanced fluorophore [25] , [26] . This achieved the sensitivity to measure kinase activity from an amount of bulk-level cell lysate estimated to be equivalent to a few cells’ worth. To perform this assay directly on a single cell selected from an adherent cell population, however, requires development of the novel capability to selectively lyse an individual adherent cell, and capture its contents while limiting dilution to retain assay sensitivity. Such a capability would open up the sensitivity, throughput and automation advantages conferred by microfluidics to a host of biochemical assays and enable their use at the single-cell level while retaining the ability to integrate these measurements with existing data from standard assay platforms. In the current work, we have developed an integrated microfluidic probe device that assays the contents of single adherent cells from standard tissue culture. It achieves selective single-cell lysis by hydrodynamic confinement of a lysis buffer at its tip and captures the contents of single cells and mixes them with assay reagents in nanolitre scale integrated chambers to perform high sensitivity single-cell assays. We demonstrate the selective lysis and capture of the contents of single adherent cells without disrupting neighbouring cells even in near-confluent cultures. We then use the device to measure kinase and housekeeping protein activities, simultaneously or separately, directly from single hepatocellular carcinoma (HepG2) cells in adherent tissue culture. We demonstrate that this approach can characterize biological heterogeneity in Akt kinase activity levels among cells under insulin stimulation. Device design and operation The integrated microfluidic probe, shown as a schematic in Fig. 1a , consists of a tip for cell lysis and collection, a region for sub-division of lysate and mixing with assay buffer, and reaction chambers controlled by pneumatic valves. The fabricated PDMS probe is shown in Fig. 1b . 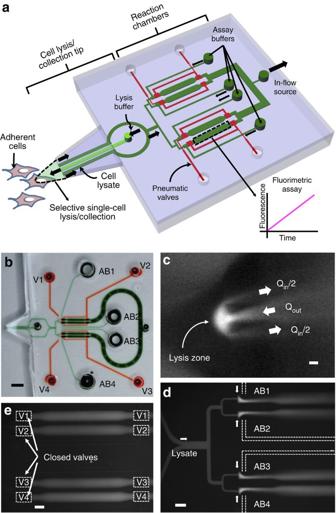Figure 1: Microfluidic probe design and operation. (a) Schematic of probe. Block arrows indicate fluid flow. (b) Fabricated PDMS device: thick top layer with channels and chambers (green), and lower thin membrane layer forming the base of the deformable tip and containing the valve lines (red, labelled V1–V4). Multiple reservoirs for assay buffers (labelled AB1–AB4) enable assaying separately for multiple activities. (c) Lysis zone is formed at tip by simultaneous in and outflows (Qinand Qout, respectively) of fluorescent lysis buffer. (d) Cell lysate can be divided and mixed with each assay buffer separately. (e) Valves are used to trap reaction mixture in chambers. Scale bars, 4 mm (b), 5 μm (c) and 200 μm (d,e). Figure 1: Microfluidic probe design and operation. ( a ) Schematic of probe. Block arrows indicate fluid flow. ( b ) Fabricated PDMS device: thick top layer with channels and chambers (green), and lower thin membrane layer forming the base of the deformable tip and containing the valve lines (red, labelled V1–V4). Multiple reservoirs for assay buffers (labelled AB1–AB4) enable assaying separately for multiple activities. ( c ) Lysis zone is formed at tip by simultaneous in and outflows (Q in and Q out , respectively) of fluorescent lysis buffer. ( d ) Cell lysate can be divided and mixed with each assay buffer separately. ( e ) Valves are used to trap reaction mixture in chambers. Scale bars, 4 mm ( b ), 5 μm ( c ) and 200 μm ( d , e ). Full size image The probe tip contains three microchannels used to create a lysis zone ( Fig. 1c ) by hydrodynamic confinement [27] , [28] , using a simultaneous outflow and inflow of lysis buffer controlled by syringe pumps (Methods). The flow rates (Q out : central channel, Q in : outer channels) are set such that in the lysis zone, convection is fast enough to prevent diffusion of molecules of interest out of the zone, as observed in a simulation of fluid flow and species transport equations using COMSOL Multiphysics ( Fig. 2a ). The size of the zone (R) is set by the separation between the outer microchannels (L), and can be further tuned using the ratio of the flow rates ( Fig. 2b ), subject to an upper bound that depends on the diffusivity of the molecule transported. The zone size is set to be slightly smaller than the diameter of the cell (~15 μm here) to allow lysis of only a single targeted cell near the probe tip. Confinement of the lysis agent to the zone ensures that neighbouring cells are not lysed, while confinement of the released lysate allows its capture back into the device. 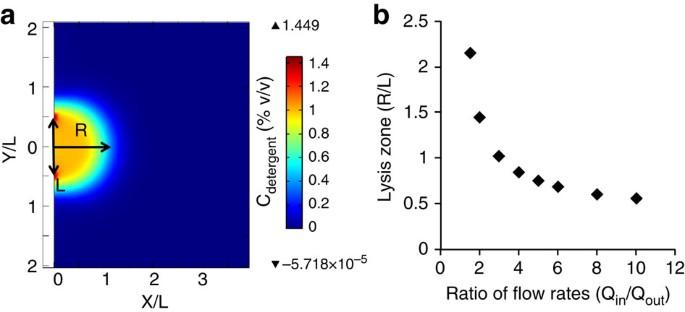Figure 2: Simulation of tunable lysis zone. (a) Plot of detergent concentration on a flat surface near the tip of the microfluidic probe, obtained from COMSOL Multiphysics simulation of fluid flow and species transport equations. The formation of a lysis zone with a high detergent concentration (1% v/v) is evident, as well as the fact that the detergent remains confined to this zone and the rest of the surface sees no detergent at all. (b) Variation of the lysis zone radius (R) with the ratio of lysis buffer outflow rate (Qout) to the lysate inflow rate (Qin)—measured as the distance from the tip at which the detergent concentration falls to 0.1%–normalized to the characteristic length scale of the tip (chosen asL=w+2p, wherewis the width of the channel, andpis the separation between channels). (For the simulation in (a),w=100 μm,p=50 μm). Figure 2: Simulation of tunable lysis zone. ( a ) Plot of detergent concentration on a flat surface near the tip of the microfluidic probe, obtained from COMSOL Multiphysics simulation of fluid flow and species transport equations. The formation of a lysis zone with a high detergent concentration (1% v/v) is evident, as well as the fact that the detergent remains confined to this zone and the rest of the surface sees no detergent at all. ( b ) Variation of the lysis zone radius (R) with the ratio of lysis buffer outflow rate (Q out ) to the lysate inflow rate (Q in )—measured as the distance from the tip at which the detergent concentration falls to 0.1%–normalized to the characteristic length scale of the tip (chosen as L = w +2 p , where w is the width of the channel, and p is the separation between channels). (For the simulation in ( a ), w =100 μm, p =50 μm). Full size image The captured single-cell lysate is pulled into the device by flow along the outer microchannels ( Fig. 1d ). The multiple chambers on the chip allow either assaying multiple cells in parallel, or performing multiple assays on a single cell. Pneumatic valves are used to direct the lysate toward a selected chamber or, optionally, to split the lysate flow into multiple parts directed toward separate chambers. Individual lysate flows are mixed with assay buffers before entering the reaction chambers ( Fig. 1d ). Lysate and assay buffer are mixed at a desired ratio determined by the ratios of flow resistances of the lysate and assay buffer microchannels ( Fig. 1d ). Lysate division and mixing ratios and the times for transport and mixing were measured, and the repeatability of each was verified to be within 10% (CV) ( Supplementary Fig. 1 , Supplementary Table 1 and Supplementary Note 1 ). The measured travel time from the tip to the reaction chamber is used to actuate the valves to capture the assay mixture ( Fig. 1e ) without requiring direct visualization of flows in the chip during the lysis, mixing and capture. The captured assay mixture can then be monitored for a readout of interest, for example, for fluorescence or absorbance by placing the chip on the microscope stage. The integration of cell lysis, mixing and assay in the microfluidic probe limits dilution of the cell lysate in this process, yielding the high sensitivity required to perform single-cell analysis. Single-cell lysis Single cells were lysed without disrupting neighbouring cells ( Fig. 3a ), even when other cells were in contact with the target cell in a relatively confluent (~80%) culture. This was verified here by monitoring fluorescence of a cytosolic dye in individual cells during the lysis process ( Fig. 3b ). Lysis of the target cell occurred immediately after exposure to the lysis zone ( Supplementary Movie 1 ), and the measured fluorescence of the target cell reduced quickly as the labelled cytosol was captured into the device, in this case, within ~20 s after lysis. The fluorescence measured from the neighbouring cells remained constant (beyond global fluctuations caused by light scattering from the placement and retraction of the tip). The repeatability and efficiency of lysis and lysate capture were characterized as shown in Supplementary Figs 2 and 3 and Supplementary Note 2 . 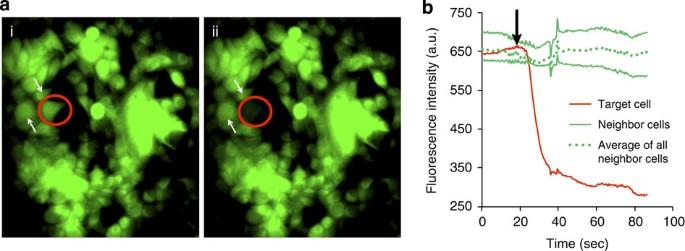Figure 3: Single-cell lysis. (a) MCF7 cells labelled with Cell Tracker Green dye are shown before (i) and after (ii) lysis of a single cell. The targeted cell is marked by a circle and several neighbouring cells are indicated by white arrows. Scale bar, 10 μm (b) Monitoring dye fluorescence in the vicinity of the targeted cell shows that lysis occurs rapidly and does not affect neighbouring cells. Note that the zero point on the time axis represents the start of imaging, while the black arrow represents the time at which the cell is exposed to lysis buffer. Traces for individual neighbouring cells correspond to cells indicated by white arrows in the figure. The dashed line represents the average fluorescence for all cells immediately bordering the target cell. Some fluctuations in signal due to retraction of the tip at time 40 s can be seen in all traces. Figure 3: Single-cell lysis. ( a ) MCF7 cells labelled with Cell Tracker Green dye are shown before (i) and after (ii) lysis of a single cell. The targeted cell is marked by a circle and several neighbouring cells are indicated by white arrows. Scale bar, 10 μm ( b ) Monitoring dye fluorescence in the vicinity of the targeted cell shows that lysis occurs rapidly and does not affect neighbouring cells. Note that the zero point on the time axis represents the start of imaging, while the black arrow represents the time at which the cell is exposed to lysis buffer. Traces for individual neighbouring cells correspond to cells indicated by white arrows in the figure. The dashed line represents the average fluorescence for all cells immediately bordering the target cell. Some fluctuations in signal due to retraction of the tip at time 40 s can be seen in all traces. Full size image Single-cell activity measurements We used the microfluidic probe to measure protein activity from single cells, employing peptide Sox sensors to monitor kinase activity, or assaying NADH formation to monitor glyceraldehyde 3-phosphate dehydrogenase (GAPDH) activity. Appropriate assay buffers (see Methods) were loaded into the reservoirs on the probe, with the flow resistances set to mix the lysate with the assay buffer at 1:4 ratio. The assay mixture was trapped in chambers and imaged over time for fluorescence. We observed fluorescence intensity increases indicating activity of the kinase Akt ( Fig. 4a ) or the housekeeping protein GAPDH ( Fig. 4b ) from single HepG2 cells. Activity values were obtained by fitting for the initial slope of such fluorescent reaction product formation traces for each cell. We observed increased Akt activities for insulin-treated cells versus serum-starved cells, as illustrated in Fig. 4a with traces from four cells. This is consistent with the expected effect of insulin treatment to stimulate Akt activity. 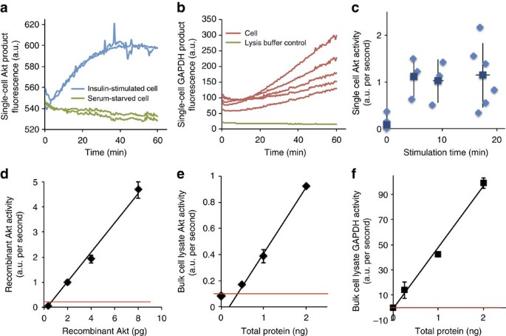Figure 4: Single-cell enzyme activity measurements. (a,b) Raw traces of reaction product fluorescence for (a) Akt for four individual HepG2 cells, two stimulated with insulin for 10 min (blue) and two unstimulated (green), and (b) GAPDH for five individual HepG2 cells. Control reaction containing no lysate is shown in (green). (c) Single-cell Akt activity values (light blue diamonds), obtained by fitting for the slope of the initial linear region of fluorescence traces, over a time course of insulin stimulation. Each point represents one cell. Mean (dark blue rectangles) and s.d. of single cell activity values are shown overlaid. (d) Calibration curve for recombinant active Akt using the device. (e,f) Calibration curves measuring bulk HepG2 lysate on the device for (e) Akt and (f) GAPDH, showing that measurement from less than half a cell’s worth of total protein is within the limit of detection of the assay (indicated approximately by the red line (mean+3s.d.)). Error bars represent s.d. Data points represent the average of two or more measurements. Figure 4c shows a time course of Akt activation by stimulation with insulin. Comparing these single-cell results (light blue diamonds) with Akt activation profiles obtained in a traditional bulk assay ( Supplementary Fig. 4a ), a similar overall trajectory is observed for the mean values (dark blue rectangles) of the single-cell measurements. The single-cell activity measurements, however, show much greater variation, particularly at later time points ( Fig. 4c and Supplementary Fig. 4b ). These fluctuations are beyond the measured technical error of this activity measurement ( Fig. 4d and Discussion below). The single-cell measurements therefore likely reflect biological variation between individual cells that is not visible in the bulk-level assay. Figure 4: Single-cell enzyme activity measurements. ( a , b ) Raw traces of reaction product fluorescence for ( a ) Akt for four individual HepG2 cells, two stimulated with insulin for 10 min (blue) and two unstimulated (green), and ( b ) GAPDH for five individual HepG2 cells. Control reaction containing no lysate is shown in (green). ( c ) Single-cell Akt activity values (light blue diamonds), obtained by fitting for the slope of the initial linear region of fluorescence traces, over a time course of insulin stimulation. Each point represents one cell. Mean (dark blue rectangles) and s.d. of single cell activity values are shown overlaid. ( d ) Calibration curve for recombinant active Akt using the device. ( e , f ) Calibration curves measuring bulk HepG2 lysate on the device for ( e ) Akt and ( f ) GAPDH, showing that measurement from less than half a cell’s worth of total protein is within the limit of detection of the assay (indicated approximately by the red line (mean+3s.d.)). Error bars represent s.d. Data points represent the average of two or more measurements. Full size image To determine the potential sensitivity of the assay, we first measured recombinant active Akt at known concentrations on both the device ( Fig. 4d ) and standard plate reader platform ( Supplementary Fig. 5 ). We established a limit of detection of 0.32 pg active Akt for the device, compared with a limit of detection of 0.51 ng active Akt on the plate reader ( Fig. 4d and Supplementary Fig. 5 ). To assess technical error and sensitivity of measurements made from cell lysate, we used the device to assay Akt activity from dilutions of bulk lysate from HepG2 cells stimulated with insulin for 20 min ( Fig. 4e ). We estimated the equivalent of a single cell’s worth of lysate as ~1 ng of total protein (Methods). The Akt activity of 0.5 ng of bulk lysate total protein could be distinguished from the no-lysate control. We also measured bulk lysate from cells stimulated with insulin for varying times and showed the ability to resolve the resulting varying Akt activities using the device ( Supplementary Fig. 6 ). An analogous calibration for the kinase MK2 yielded a similar limit of detection ( Supplementary Fig. 7 ). The limit of detection for GAPDH was even lower ( Fig. 4f ), likely due to greater expression levels of GAPDH relative to Akt. The Akt activity of 1 ng of diluted bulk lysate compared reasonably (approximately fourfold lower) with values obtained for the single-cell assay. For GAPDH, the bulk activity values were higher than the single-cell values. This could be because of slight temperature or pH differences owing to the presence of medium in the reaction in the single-cell case. On average, the coefficient of variation for Akt bulk lysate measurements was within 7%, and the analogous number for GAPDH bulk lysate measurements was within 18%. The observed limits of detection correspond to fractions of the total protein content of a single cell, suggesting sufficient sensitivity to allow multiplexed enzyme activity measurement from single cells. To measure Akt and GAPDH activity simultaneously from individual cells, lysate from a single cell was subdivided and mixed with separate assay buffers and collected in separate chambers. Using this approach, we measured both activities from single serum-starved and insulin-stimulated cells. We observed that for some cells, Akt activity increased as expected upon stimulation with insulin, whereas GAPDH activity was unaffected by this treatment, as shown in Fig. 5a (dark blue and dark red markers). However, for a subset of cells, GAPDH activity was present while Akt activity was not ( Fig. 5a , light blue and light red markers). 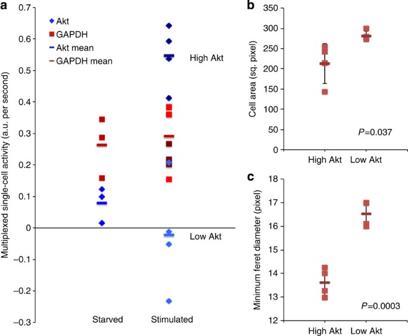Figure 5: Multiplex single-cell enzyme activity measurements. (a) Measurements of Akt (blue) and GAPDH (red) activity simultaneously from single cells (n=12). For ‘high Akt’ cells, Akt activity (dark blue) increases upon stimulation with insulin for 16.5 min (P-value of 3.2 × 10−4), whereas GAPDH activity (dark red) is unaffected (P-value of 0.98). For ‘low Akt’ cells, neither Akt (light blue) or GAPDH (light red) activities are affected by insulin stimulation (P-values of 0.35 and 0.50, respectively). The negative values indicate that these measured slopes were lower than the lysis buffer control value, which reflects an increased contribution from photobleaching. (b,c) Statistically significant differences are seen between ‘high Akt’ and ‘low Akt’ cells in the morphological parameters of (b) cell area and (c) minimum Feret diameter (or caliper width) (P-values for Student’st-tests as shown). Error bars represent s.d. Figure 5: Multiplex single-cell enzyme activity measurements. ( a ) Measurements of Akt (blue) and GAPDH (red) activity simultaneously from single cells ( n =12). For ‘high Akt’ cells, Akt activity (dark blue) increases upon stimulation with insulin for 16.5 min ( P- value of 3.2 × 10 −4 ), whereas GAPDH activity (dark red) is unaffected ( P- value of 0.98). For ‘low Akt’ cells, neither Akt (light blue) or GAPDH (light red) activities are affected by insulin stimulation ( P- values of 0.35 and 0.50, respectively). The negative values indicate that these measured slopes were lower than the lysis buffer control value, which reflects an increased contribution from photobleaching. ( b , c ) Statistically significant differences are seen between ‘high Akt’ and ‘low Akt’ cells in the morphological parameters of ( b ) cell area and ( c ) minimum Feret diameter (or caliper width) ( P- values for Student’s t- tests as shown). Error bars represent s.d. Full size image Examining these two groups of cells revealed morphological differences between them. Relative to cells that exhibited higher Akt activity in response to insulin stimulation (‘high Akt’), the cells that did not respond in this way to insulin stimulation (‘low Akt’) were significantly larger in cell area as well as in minimum Feret diameter, a measure of cell width ( Fig. 5b,c ). In support of the relevance of these morphological observations, the measured cells’ values fall within the overall distribution of the minimum Feret diameter for a larger number of cells out of the HepG2 population under these conditions ( Supplementary Fig. 8 ). In addition, the shape of this overall distribution appears consistent with the existence of multiple morphological subtypes ( Supplementary Fig. 8 ). Thus, this device enabled the identification of two subgroups of cells from a population in tissue culture with differences in signalling that corresponded to differences in cell phenotype. We have shown that the microfluidic probe can be used to lyse an individual adherent cell without disrupting neighbouring cells, even from a fairly confluent plate, using hydrodynamic confinement. This is, to our knowledge, the first use of hydrodynamic confinement to reclaim cellular material for assay. The integration of all steps in the lysis, mixing and assay process in a single chip limits lysate dilution at each step and maintains the assay mixture within a nanolitre volume, making it possible to use standard biochemical assays at single-cell sensitivity. We applied the microfluidic probe to measure kinase activity, since direct activity measurements present a significant advantage over indirect signalling readouts but are more challenging using current single-cell methods. In this case, using the current device, two to four activities can be measured from a given cell. This provides the opportunity not only for multiple readouts of interest from a single cell, but also for the normalization of measured activities to a reference readout (loading control) as another way to address technical variability. GAPDH is commonly used as a loading control for experiments measuring protein or mRNA levels. A characterization of the distribution of GAPDH activities across a cell population of interest would be desirable for its use as a loading control on a per cell basis, which would be possible using our device. Here, dividing the Akt (‘high Akt’) measurements by the corresponding GAPDH measurement for each individual cell, we see a very similar pattern of response to insulin stimulation ( Supplementary Fig. 9 ). Combinations other than the one we chose (Akt and GAPDH) are a possibility, given the existence of Sox sensors for a panel of kinases, including Akt, Erk1/2, PKA, MK2 and p38α [25] , [29] , [30] , representing a variety of signalling pathways, and the fact that the GAPDH assay used here simply monitors conversion of NAD + to the fluorescent molecule NADH and thus represents a method generally applicable for numerous metabolic enzymes. Because this platform provides a general way to access the lysate from a single adherent cell, it can therefore, in principle, also be combined with other types of assays–for example, to assay gene expression, or obtain other readouts directly from single cells in a context of interest. The device can be optimized to obtain even higher sensitivity for biochemical assays by reducing the assay volume (currently 20 nl), which would also enable further multiplexing. Further sensitivity increases could be achieved by integration with a microfluidic concentrator [31] . Currently, the device can be used to assay four cells in parallel. While multiple reaction mixtures can be assayed simultaneously, cell lysis and collection are currently performed separately for each cell. Parallelizing and automating this process, and increasing the number of chambers, will help to improve the throughput. Such technical improvements are well within the realm of current microfluidics technology. The current throughput, however, is expected to be sufficient for a number of biological applications. Levels of many proteins and mRNA transcripts in mammalian cells have been observed to follow a log-normal distribution with a biological coefficient of variation of 15–30% [3] , [32] , [33] , [34] . We conducted simulations ( Supplementary Figs 10 and 11 and Supplementary Note 3 ) to determine, given the technical error of measurement on the device, the number of measurements required to statistically distinguish two subpopulations of cells (identified, for example, by a phenotypic characteristic such as morphology) with respect to a particular measured level. These results indicated that for a conservative biological coefficient of variation of 30%, on the order of tens of measurements were sufficient to resolve the two subpopulations, even when their means differed by as little as 30% ( Supplementary Table 2 and Supplementary Note 3 ). The ability of the probe to access single cells from adherent tissue culture makes it compatible with standard phenotypic assays performed in these platforms, meaning that the probe could be used along with such assays in order to obtain multiple types of information from the same cells. Indeed, in a pilot study, we identify two subsets of HepG2 cells under insulin stimulation with respect to Akt activity, which we term ‘low Akt’ and ‘high Akt’ cells, and identify statistically significant differences in morphology between them. The measured parameters of the ‘low Akt’ cells are consistent with a wider, flatter morphology, changes that are observed in HepG2 cells undergoing cellular senescence [35] , [36] . There is evidence that Akt activity may be lower during senescence [37] , [38] , and in HepG2 cells, SMP-30, a marker that is low in senescence, promotes Akt activity, consistent with lower Akt activity in senescent HepG2 cells [39] . Indeed, a senescence-associated beta-galactosidase (SA-β-gal) assay revealed increased SA-β-gal activity under the conditions of this single-cell assay (sparsely plated) relative to a negative control (higher density), up to the level of a positive control (doxorubicin treatment) ( Supplementary Fig. 12 , Supplementary Table 3 and Supplementary Note 4 ). Thus, the observed morphology differences, which correlate with Akt activity level, could be related to senescence, suggesting an avenue for further investigation into the existence of these two subpopulations of cells. While this aspect of the study remains preliminary, it illustrates the potential of this assay approach for connecting signalling measurements with cellular phenotypes in their relevant context. The altered morphology phenotype would not be possible to observe in flow cytometry assays, for example, and this probe allows us to select wider, flatter cells versus normal cells individually and specifically examine signalling in each. The use of the probe with standard tissue culture platforms also facilitates the comparison of probe-based measurements to measurements made in traditional bulk assays. Thus, this platform provides the potential to directly match multiplexed biochemical measurements with contextual or phenotypic information (for example, from standard assays for morphology, migration or invasion) for the same individual cell, helping to clarify the connections between intracellular states and cellular outcomes. In addition, the ability to use the probe with non-genetically modified adherent cells affords the significant advantage of making it potentially usable with primary cells and tissue sections. These features will make the device useful in the investigation of heterogeneity in cell populations, with particular relevance to situations where a few phenotypically distinct cells are of interest but are difficult to isolate for investigation. For example, tumour cell invasion and metastasis are processes of great therapeutic import that are marked by heterogeneity [1] , and studies to determine what makes a few cells capable of invading away from a tumour have been hampered by difficulties in accessing and assaying these few cells [40] . The method presented here would allow such cells to be examined individually. Lysis zone simulations Two-dimensional simulations of detergent concentration in and outside the lysis zone were conducted using COMSOL Multiphysics. Fluid flow was simulated at various inflow (Q in ) and outflow (Q out ) rates using the Laminar Flow module ( spf ), using the fluid properties of water. The flow velocity profile obtained was then used as input to the Transport of Dilute Species module ( chds ) to simulate the convection and diffusion of the detergent, using a detergent diffusivity of 6 × 10 −11 m 2 s −1 and an input concentration of 1% (V/V). The radius of the lysis zone (R) was obtained from the simulated detergent concentration profile, as the distance from the tip at which the detergent concentration falls to 0.1%. The variation of this radius with flow rate ratio was then examined. Microfluidic device design and fabrication The microfluidic probe ( Fig. 1b ) consists of three layers: a bare glass slide that forms the base except at the tip, a thin PDMS membrane (~30 μm) layer that forms the base of the tip and enables the probe to reach close to adherent cells and also contains the pneumatic valve lines, and a thick (~5 mm) flow layer that contains the channels, chambers and flow and control connection ports. The flow layer itself has channels of two different heights: 5 μm tall channels for the tip and assay buffer mixing regions that are designed to ensure 1:4 mixing (by tuning the flow resistance ratio) and the 30 μm tall reaction chambers that maximize fluorescence sensitivity. The PDMS layers were made and thermally bonded together by standard two-layer soft lithography methods [41] . Briefly, a mask pattern drawn in AutoCAD 2000 and transferred to a photoplot film or a chrome mask was used for photolithography to create two photoresist moulds on standard 6 inch silicon wafers: the flow-layer mould using AZ4620 for the 30 μm tall channels and SU-8 for the 5 μm flow channels, and the membrane-layer mould using SU-8 for the 15 μm valve lines. The masters were silanized by placing both inside dessicators, each with a drop of Heptadecafluoro-1,1,2,2-tetra-hydrodecyl trimethoxysilane, venting the dessicators for 1 min, then maintaining the vacuum for 1 h. A thin layer of mixed, degassed PDMS (RTV615, 20:1) was spin-coated at 1,600 r.p.m. on the membrane-layer mould. A thicker layer of PDMS (5:1) was poured on the flow-layer mould. For this layer, after initial casting from the silicon mould, a plastic replica of the mould was created for further use [42] . Both PDMS layers were partially cured for 60 min at 65 °C. The thicker flow-layer PDMS was then peeled from its mould and aligned to the membrane layer on its mould under a stereo microscope and brought into contact with it. After ensuring bubble-free contact, the mould was baked overnight at 65 °C to obtain monolithic devices. The cured monolithic PDMS piece with channels and valves was cut and peeled from the flow-layer mould and access holes were punched into it using a biopsy punch. The tip region of the cured PDMS device was cut with a sharp microtome blade to have a pointed tip with a flat front. The PDMS device and a glass slide were exposed to plasma and brought into contact such that only the tip region protruded over a straight edge of the glass. The assembled device was baked at 95 °C for 15 min and then degassed for at least 10 min before use. Device preparation Devices were prepared for use by priming the channels with de-ionized water using gas-tight glass syringes (50 μl) connected to the lysis buffer and inflow source ports ( Fig. 1a ) using fused silica tubing (OD: 360 μm, ID: 100 μm). Devices were coated with bovine serum albumin (BSA) to prevent non-specific protein binding to PDMS surfaces by drawing in a 1% solution of BSA in 0.5 × phosphate-buffered saline under a small flow rate (50 nl min −1 ) maintained using syringe pumps (Harvard Apparatus, PHD 2000) for at least 1 h and then washed with de-ionized water. The area of the device observed during the assay was bleached for at least 30 min using ultraviolet light ( λ ex =377 nm) before use to reduce background fluorescence. Immediately before use, lysis buffer was loaded into the syringe connected to the lysis buffer port, and assay buffer(s) were loaded into the appropriate assay buffer reservoirs (20 μl each). Cell culture, labelling and stimulation HepG2 cells (ATCC, HB-8065) were grown on tissue culture treated polystyrene at 37 °C and 5% CO 2 , using Eagle’s Minimal Essential Medium supplemented with 10% fetal bovine serum (Hyclone, Fisher Scientific) and 1% penicillin/streptomycin (Invitrogen). Cells were labelled with Cell Tracker Orange dye (Invitrogen) by incubating serum-starved cells with 2.5 μM Cell Tracker dye in serum-free medium for 15–45 min at 37 °C and 5% CO 2 . Cells were washed with phosphate-buffered saline and allowed to recover in serum-free medium at 37 °C and 5% CO 2 for 20–45 min before the start of an experiment. Stimulations were conducted either by spiking in an appropriate concentration of reagent, or by replacing the medium with serum-free medium containing the desired reagent concentration (500 ng ml −1 insulin final) on cells that had been serum starved for 12–24 h. At the desired treatment time point, medium was removed and cells were immediately washed and placed in serum-free medium. The plate was then brought to the device setup and the lysis procedure started immediately. For time courses using the device, medium containing the stimulation condition was not removed and cells were lysed one by one off the plate under stimulation conditions using the device. Buffer conditions Lysis buffer contained 50 mM β-glycerophosphate, 10 mM sodium pyrophosphate, 30 mM sodium fluoride, 50 mM Tris buffer, pH 7.4; 1% Triton X-100 detergent, 15 mM NaCl, 2 mM EGTA, 100 μM sodium orthovanadate, 1 mM DTT, and 1X protease and phosphatase inhibitor cocktails (Merck/EMD 539134 and Sigma P2850, respectively). A quantity of 20 μg ml −1 Alexa 488-labelled BSA was added to the lysis buffer to allow visualization of the lysis zone outside the microfluidic probe tip. Kinase activity assay conditions were 50 mM Tris-HCl (pH 7.3), 10 mM MgCl 2 , 1 mM EGTA, 2 mM DTT, 4 μM PKC inhibitor peptide, 10 μM substrate peptide, 1 mM ATP (low metals grade; Calbiochem), 0.4 μM PKItide, and 5 μM and 25 μM GF109203X (EMD) for Akt and MK2, respectively (as in Shults et al. [25] , except without the inclusion of calmidazolium, as it was observed to cause problems in the device, possibly from surface binding). GAPDH activity assays were conducted in 90 mM sodium pyrophosphate, pH 7.1, 20 mM NaH 2 PO 4 , 3 mM DTT, 4 mM NAD + and 10 mM glyceraldehyde 3-phosphate. Single-cell lysis and assay procedure Briefly, HepG2 cells were plated at 5–20,000 cells per cm 2 on standard tissue culture plastic and allowed to attach for 4–16 h, then serum starved overnight. Cells were labelled with Cell Tracker Orange dye, then stimulated to activate the kinase of interest. Following stimulation, the plate was placed on the microscope (Olympus IX71) and the microfluidic probe was positioned near the cell of interest using a micromanipulator. The lysis zone was created by starting the outflow of lysis buffer (5 nl min −1 ), while maintaining inflow through the device of 50 nl min −1 . This is expected to result in a local flow at each of the outer channels of the tip of 5 nl min −1 . Inflow and outflow of lysis buffer were each controlled by a separate syringe pump. Cell lysis was observed by imaging for Cell Tracker Orange fluorescence using a rhodamine filter (Semrock, λ ex =540 nm, λ em =570 nm). Lysate flowing into the chip mixes with assay buffer, and taking into account the appropriate amount of travel time for fluid flow through the device (90 s), valves were actuated using compressed air (30 psi) supplied through a custom-built manifold with solenoid valves to trap this assay mixture in chambers on the device. For observation of the assay chambers over time, the chip was placed on the microscope at 30 °C in a heating chamber (Tokai Hit) on an automated motorized stage (Prior Scientific, H110). Fluorescence intensity was monitored by imaging sensor fluorescence using a DAPI filter (Semrock, λ ex =377 nm, λ em =447 nm) every 30 s using a shutter (Vincent Associates, Uniblitz) for at least twenty minutes at an exposure of 200 ms, to observe conversion of the substrate to fluorescent product by the enzyme of interest. Images were quantified using ImageJ. The slope of the initial increase in fluorescence intensity was taken to represent the activity of the kinase. Activity values were corrected for bleaching by subtracting the mean of the lysis buffer control reaction. Statistical significance was determined using a two-tailed t -test with unequal variances, in Excel. Cell morphology quantification Cell morphology was quantified using ImageJ. Statistically significant differences were determined as above. Bulk stimulation, lysis and kinase assay HepG2 cells were stimulated for kinase activity and lysed as previously described [25] . Briefly, cells were seeded at 15–100,000 cells per cm 2 on standard tissue culture plastic and allowed to attach overnight. No changes in insulin activation time course were seen for seeding densities within this range (data not shown). Cells were serum starved for 16–24 h, then stimulated to activate the kinase of interest (by spiking in to a final concentration 500 ng ml −1 insulin to activate Akt, or replacing the medium with 300 mM sorbitol in serum-free medium to activate MK2). At the desired time point, cells were washed and lysed on ice via scraping and the lysis buffer described above. Lysates were clarified, aliquotted and flash frozen in liquid N 2 . Kinase activity assays were carried out in 50 mM Tris-HCl (pH 7.3), 10 mM MgCl 2 , 1 mM EGTA, 2 mM DTT, 0.1% Brij-35, 4 μM PKC inhibitor peptide (EMD), 10 μM substrate peptide, 1 mM ATP (low metals grade; EMD), 0.4 μM PKItide (EMD) and 5 μM and 25 μM GF109203X (EMD) for Akt and MK2, respectively [25] using a plate reader (M2e, SpectraMax) and half-volume 96-well plates (Corning, 3992). We estimated the equivalent of a single cell’s worth of lysate as ~1 ng of total protein based on cell counts and total protein measurements from bulk assays. For example, lysis of a well containing ~400,000 HepG2 cells resulted in recovery of 360 μg of total protein. How to cite this article : Sarkar, A. et al. Microfluidic probe for single-cell analysis in adherent tissue culture. Nat. Commun. 5:3421 doi: 10.1038/ncomms4421 (2014).